Louisville seamount subduction and its implication on mantle flow beneath the central Tonga–Kermadec arc Subduction of intraplate seamounts beneath a geochemically depleted mantle wedge provides a seldom opportunity to trace element recycling and mantle flow in subduction zones. Here we present trace element and Sr, Nd and Pb isotopic compositions of lavas from the central Tonga–Kermadec arc, west of the contemporary Louisville–Tonga trench intersection, to provide new insights into the effects of Louisville seamount subduction. Elevated 206 Pb/ 204 Pb, 208 Pb/ 204 Pb, 86 Sr/ 87 Sr in lavas from the central Tonga–Kermadec arc front are consistent with localized input of subducted alkaline Louisville material (lavas and volcaniclastics) into sub-arc partial melts. Furthermore, absolute Pacific Plate motion models indicate an anticlockwise rotation in the subducted Louisville seamount chain that, combined with estimates of the timing of fluid release from the subducting slab, suggests primarily trench-normal mantle flow beneath the central Tonga–Kermadec arc system. Sites of plate convergence (subduction zones) have a key role in material recycling on Earth. A volcanic arc is the surface expression of subduction-accompanied dehydration and partial melting processes at depth. During dehydration at higher pressures, hydrous fluids are expelled from the subducting slab (consisting of sediment cover, altered oceanic crust and serpentenized uppermost lithosphere) into the overlying mantle wedge. This lowers the mantle solidus, resulting in partial melting. Arc lavas commonly carry signals of these fluids, which could be either aqueous fluids or supercritical fluids and melts (for example, refs 1 , 2 , 3 ). There is some consensus among researchers concerning the transfer of elements via fluids from the subducting slab and partial melting of the overlying mantle wedge, but there is debate regarding the geometry of mantle flow in the wedge. Classical mantle corner flow models invoke trench-normal flow geometry in the mantle wedge, a hypothesis supported by seismic anisotropies observed in the Izu Bonin arc [4] . Conversely, trench-parallel mantle flow has been suggested beneath the Central American Arc [5] and Vanuatu Arc [6] , based on both seismic anisotropy measurements and arc geochemical signatures. Trench-parallel seismic anisotropies identified along the northern Tonga arc [7] , [8] have been interpreted as reflecting rapid, along-arc southward mantle flow, consistent with the inflow of Indo-Australian mantle replacing Pacific mantle along the northern Lau Basin [9] . Since ~4 Ma, the Louisville seamount chain on the Pacific Plate is believed to have undergone subduction beneath the Indo-Australian plate. Assuming a consistency in azimuth between the unsubducted and subducted portion of the Louisville seamount chain, the obliquity between the unsubducted chain azimuth and the convergence azimuth suggests a net southward migration of the collision zone [10] . Geochemical data from the Tonga and northern Kermadec arc show a depleted MORB-type mantle wedge composition (for example, refs 11 , 12 ). This composition should be highly sensitive to contamination by enriched components, such as alkaline Louisville seamount material (for example, refs 13 , 14 , 15 ), making this an ideal region in which to study material recycling from the subducting slab, and mantle wedge flow geometry. Here, we present evidence for the existence of a radiogenic isotope signature derived from subducting Louisville seamount chain rocks in recent lavas (<10 ka) from the central Tonga–Kermadec arc volcanic centers ‘U’, ‘V’ and Monowai, and the southern Lau back arc and older lavas (<100 ka) from Ata Island (hereafter collectively named central Tonga–Kermadec arc). All of these sites are located near the contemporary point of collision between the Louisville seamount chain and the Tonga–Kermadec trench. Geochemical evidence is complemented by analyses of seismicity and forearc morphology, which in addition to plate reconstruction models support previous suggestions [16] of an alternate more westerly geometry for the subducted portion of the Louisville seamount chain. Geological and geochemical background Located in the southwest Pacific ocean, the ~2,600-km-long Tonga–Kermadec arc is the most linear, fastest converging and most seismically active subduction boundary on Earth (for example, ref. 17 ; Fig. 1 ). This collision zone between the Pacific and Indo-Australian tectonic plates is characterized by one of the world’s deepest trenches and the most volcanically active arc, with the highest density of submarine volcanic centers (>1 per 50 km of strike) [18] . At ~25.4°S the Tonga–Kermadec trench is intersected by the Louisville Ridge, a ~4,300-km-long chain of seamounts and guyots, which formed over the past 80 Myr as the Pacific Plate passed over a hotspot presently located near the intersection of the Eltanin Fracture Zone and the East Pacific Rise [19] . This collision zone is coincident with the first-order tectonic boundary between the Tonga and Kermadec segments of the plate boundary, which exhibit significant differences in forearc morphology, subducting slab geometry, back-arc-spreading dynamics and seismicity [20] , [21] , [22] . 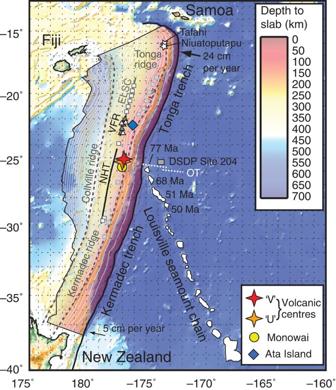Figure 1: Bathymetric map of the Tonga–Kermadec arc system. Map showing the depth of the subducted slab beneath the Tonga–Kermadec arc system (modified after USGS slab surface figure;http://earthquake.usgs.gov/research/data/slab). Louisville seamount ages are after Kopperset al.49ELSC, eastern Lau-spreading centre; DSDP, Deep Sea Drilling Programme; NHT, Northern Havre Trough; OT, Osbourn Trough; VFR, Valu Fa Ridge. Arrows mark total convergence rates17. Grey squares (named volcanic centers), white squares (Lau Basin, Havre Tough) and grey and white triangles (Valu Fa ridge and seamounts) mark sample locations. Figure 1: Bathymetric map of the Tonga–Kermadec arc system. Map showing the depth of the subducted slab beneath the Tonga–Kermadec arc system (modified after USGS slab surface figure; http://earthquake.usgs.gov/research/data/slab ). Louisville seamount ages are after Koppers et al. [49] ELSC, eastern Lau-spreading centre; DSDP, Deep Sea Drilling Programme; NHT, Northern Havre Trough; OT, Osbourn Trough; VFR, Valu Fa Ridge. Arrows mark total convergence rates [17] . Grey squares (named volcanic centers), white squares (Lau Basin, Havre Tough) and grey and white triangles (Valu Fa ridge and seamounts) mark sample locations. Full size image The Pacific plate increases in age from ~85 to 144 Ma north and south of the Osbourn trough paleo-spreading centre, respectively [23] , [24] , which, together with a ~200-m-thick sediment cover (drilled at DSDP Site 204 west of the trench, see Fig. 1 ), has been subducting beneath the Australian Plate since at least the late Oligocene (for example, ref. 25 ). The volcanic front in this region lies between ~140 km (Monowai) and ~190 km (Ata) west of the trench, 40–60 km west of the Kermadec Ridge (for example, refs 26 , 27 ) and 120–130 km above the subducting slab (average slab dip of ~30°, which steepens to ~45° beneath a depth of 120 km; Fig. 1 ) [28] . The volcanic centers ‘U’ (25.44°S; 177.11°W) and ‘V’ (25.19°S; 177.06°W) [29] are located ~320 km south of Ata, ~180 km west of the current intersection between the Tonga–Kermadec trench and the Louisville seamount chain, and ~50 km north of the atypically large mafic Monowai volcanic centre. Both were sampled during the R/V Tangaroa NZAPLUME III expedition in 2004. Sixteen 100% normalized volatile-free rock compositions from ‘U’ (8) and ‘V’ (8) range from basalt to rhyolite (49.6–71.3 wt.% SiO 2 ) [27] and belong to the low-K tholeiitic series [30] . All the lavas show typical arc-type enrichments of large ion lithophile elements (LILE; Rb, Ba, U, K, Pb, Sr), Nb depletions compared with normal mid-ocean ridge basalt (N-MORB after Sun and McDonough [31] ) and depleted- to slightly enriched-MORB-type high-field element distributions on a multi-element diagram ( Fig. 2 , Supplementary Table S1 ). Sr and Pb isotopic compositions of lavas from ‘U’, ‘V’, Monowai and Ata are generally more radiogenic than Pacific and Indian MORB ( Fig. 3 ) [12] , [32] , [33] , but their Nd isotopic compositions fall within the MORB range [34] . The Sr, Nd and 207 Pb/ 204 Pb isotopic values are similar, but the 206 Pb/ 204 Pb and 208 Pb/ 204 Pb values are more radiogenic than most other lavas sampled along the mid-Tonga to northern Kermadec arc segments. Similarly high 206 Pb/ 204 Pb and 208 Pb/ 204 Pb values are apparent in back-arc lavas from the southern Valu Fa Ridge and in seamounts east of Ata Island and the southern Lau Basin at 23.93°S ( Fig. 3 ) [32] , [35] , [36] , [37] , [38] . 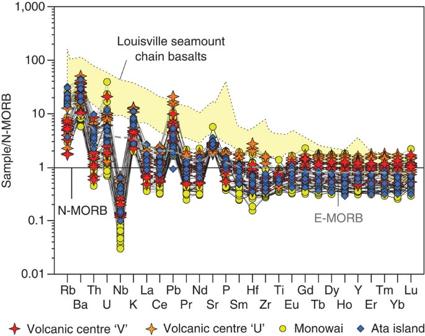Figure 2: Multi-element diagram. N-MORB normalized31multi-element diagram of the volcanic centers Monowai12, U, V (this study) and Ata26. Yellow field represents the Louisville seamount chain lavas (LSCL) after13,14,15. Grey dashed line marks average enriched mid-ocean ridge basalts (E-MORB) after Sun and McDonough31. Figure 2: Multi-element diagram. N-MORB normalized [31] multi-element diagram of the volcanic centers Monowai [12] , U, V (this study) and Ata [26] . Yellow field represents the Louisville seamount chain lavas (LSCL) after [13] , [14] , [15] . Grey dashed line marks average enriched mid-ocean ridge basalts (E-MORB) after Sun and McDonough [31] . 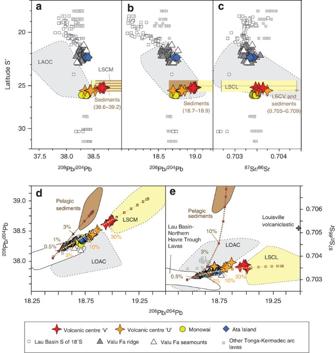Figure 3: Sr and Pb isotope data. (a) Latitude °S versus208Pb/204Pb, (b)206Pb/204Pb, (c)87Sr/86Sr, (d)206Pb/204Pb versus208Pb/204Pb and (e)206Pb/204Pb versus87Sr/86Sr. Dashed lines with squares are mixing curves between the Lau Basin-northern Havre Trough lavas, pelagic sediments (brown) and Louisville lavas (yellow). SeeSupplementary Table S2for modelling details. LAOC (local altered oceanic crust) after46,47. LSVC, Louisville seamount chain volcaniclastics (DSDP Site 204)45; LSCL, Louisville seamount chain lavas13,14,15; LSCM, Louisville seamount chain material (lavas and volcaniclastics). Sediment data are taken from Ewartet al.45Lau Basin and northern Havre Trough lavas are after32,33,37,38. Valu Fa Ridge and seamount lava data are after33,35,36,37,38. Other Tonga–Kermadec arc lava data are taken from12,33,37,45,57,58,62. As discussed in33,37,58the Pb isotope data set of Turneret al.26were affected by analytical artifacts leading to lower206Pb/204Pb values outside of the analytical error compared with new analyses on the same samples and were omitted in this compilation. For further details, the reader is referred to33,37,58. Full size image Figure 3: Sr and Pb isotope data. ( a ) Latitude °S versus 208 Pb/ 204 Pb, ( b ) 206 Pb/ 204 Pb, ( c ) 87 Sr/ 86 Sr, ( d ) 206 Pb/ 204 Pb versus 208 Pb/ 204 Pb and ( e ) 206 Pb/ 204 Pb versus 87 Sr/ 86 Sr. Dashed lines with squares are mixing curves between the Lau Basin-northern Havre Trough lavas, pelagic sediments (brown) and Louisville lavas (yellow). See Supplementary Table S2 for modelling details. LAOC (local altered oceanic crust) after [46] , [47] . LSVC, Louisville seamount chain volcaniclastics (DSDP Site 204) [45] ; LSCL, Louisville seamount chain lavas [13] , [14] , [15] ; LSCM, Louisville seamount chain material (lavas and volcaniclastics). Sediment data are taken from Ewart et al. [45] Lau Basin and northern Havre Trough lavas are after [32] , [33] , [37] , [38] . Valu Fa Ridge and seamount lava data are after [33] , [35] , [36] , [37] , [38] . Other Tonga–Kermadec arc lava data are taken from [12] , [33] , [37] , [45] , [57] , [58] , [62] . As discussed in [33] , [37] , [58] the Pb isotope data set of Turner et al. [26] were affected by analytical artifacts leading to lower 206 Pb/ 204 Pb values outside of the analytical error compared with new analyses on the same samples and were omitted in this compilation. For further details, the reader is referred to [33] , [37] , [58] . Full size image Central Tonga–Kermadec arc and back-arc geochemical variations Elevated contents of aqueous fluid-mobile elements (for example, Ba, Sr, Pb, U) and generally MORB-like contents and ratios of aqueous fluid-immobile elements (for example, (La/Sm) N <0.9; N =normalized to C1 chondrite after McDonough and Sun [39] ) [12] , [32] in Monowai, ‘U’ and ‘V’ lavas are consistent with element transfer from the subducting slab to the central Tonga–Kermadec mantle wedge via aqueous fluids [2] . Lavas from Ata, however, have elevated (La/Sm) N ≥0.9, indicating either a lower degree of partial melting, or a local source enrichment in the mantle wedge [26] . Back-arc lavas show similar elevations in (La/Sm) N , which increases from ~0.6 at the eastern Lau-spreading centre, to ≥1.0 at the southern tip of the Valu Fa ridge (for example, refs 33 , 35 , 36 , 37 ). This increase has been attributed to the north–south reduction in distance between the Valu Fa ridge and the arc front volcanoes, which reaches a minimum of ~40 km between the arc front and the southern tip of the Valu Fa Ridge [35] , and whose melts therefore may have influenced the melt genesis in the back-arc mantle (for example, ref. 33 ). A single analysis from the southernmost Lau Basin sampled at 23.9°S [32] , however, shows relatively low (La/Sm) N of ~0.6, also suggesting that local source enrichment beneath the Ata region has taken place. There are two primary explanations for the Sr and Pb isotope variability in arc lavas: (1) mantle wedge compositional heterogeneity, and (2) variable incorporation of subducted material (that is, sediment cover, altered oceanic crust and serpentenized, uppermost lithosphere) into partial melts. Although it has been proposed that the Nd and Hf isotopic compositions of northern Tonga–southern Kermadec lavas represent pre-existing mantle wedge heterogeneities (for example, refs 12 , 40 , 41 ), the corresponding Sr and Pb isotopic compositions are interpreted as reflecting slab-derived, fluid-transported Sr and Pb from altered oceanic crust and sediment cover into the overlying mantle wedge (for example, refs 42 , 43 , 44 ). This dichotomy allows us to track slab-derived inputs through the ‘subduction factory’. The slightly higher 206 Pb/ 204 Pb and 208 Pb/ 204 Pb values from Ata and Monowai compared with other mid-Tonga–Kermadec arc lavas can be explained through mixing of local pelagic sediments (as drilled at DSDP Site 204) [26] , [45] and altered oceanic crust ( Fig. 2 ) [46] , [47] with Lau Basin–Havre Trough back-arc mantle. ‘U’ and ‘V’ lavas have similar to slightly higher 206 Pb/ 204 Pb, but significantly higher 208 Pb/ 204 Pb values than local sediment plus ‘normal’ altered oceanic crust ( Fig. 3 ). These latitudinal variations in Pb isotope compositions ( Fig. 3a ) thus cannot be explained by input of pelagic sediment and/or ‘normal’ altered oceanic crust-derived Pb. Similar 207 Pb/ 204 Pb and 87 Sr/ 86 Sr values in lavas along the mid-Tonga arc north of Ata and Kermadec arc south of Monowai argue against increased aqueous fluid-transported sediment Pb and Sr input to the central Tonga–Kermadec arc lavas. Addition of Louisville components having higher 206 Pb/ 204 Pb, 208 Pb/ 204 Pb, similar to higher 87 Sr/ 86 Sr and similar 207 Pb/ 204 Pb isotope composition can explain the variation in Sr and Pb isotope compositions of Monowai, ‘U’, ‘V’ and ‘Ata’. Hence, we interpret latitudinal variations in Pb isotope compositions as reflecting the variable availability and incorporation of Pb and Sr derived from Louisville volcanic material into partial melts. Following previous results from Monowai [12] , [32] , the pre-Louisville Pb and Sr isotope composition of the mantle wedge most likely resembles that of the Lau Basin north of ~22°S, with ~0.5% fluid-derived Pb and a small Sr contribution from the subducted sediment (cf. that drilled in the upper 100 m of DSDP Site 204) (for example, refs 12 , 32 ). Assuming an average Louisville isotopic composition of 206 Pb/ 204 Pb=19.34, 208 Pb/ 204 Pb=39.04 and 87 Sr/ 86 Sr=0.70359, up to ~40% of a slab-derived Louisville signature, is required to explain the highest 206 Pb/ 204 Pb, 208 Pb/ 204 Pb and 87 Sr/ 86 Sr values for ‘V’ ( Fig. 3d ), a ~20% for ‘U’ and ~5% for Monowai, Ata and Valu Fa ( Fig. 3d ). The more radiogenic nature of Sr in volcaniclastic sediments makes it possible to discriminate between sediment- and lava-driven compositional variations. Incorporation of volcaniclastic material into the mantle source beneath the central Tonga–Kermadec arc should result in elevated Sr isotope values, which is only observed to a minor extent in lavas from ‘U’ and ‘V’. Pb and Sr each have different mobility in aqueous fluids (for example, refs 43 , 44 ) and may, therefore, be decoupled. However, as we observe only a minor increase in Sr, we favour a predominant influence through dehydration of the altered Louisville crust. The progressive increase of Ba/Th at similar 206 Pb/ 204 Pb [45] , [37] suggests that the slab-derived fluids beneath the Tonga arc have high Ba/Th (~1,200) and 206 Pb/ 204 Pb of~18.5–18.6, which, if applied to Louisville-derived fluid, would result in similarly high to even higher Ba/Th, and 206 Pb/ 204 Pb of ~19.0 can be inferred ( Fig. 4 ). 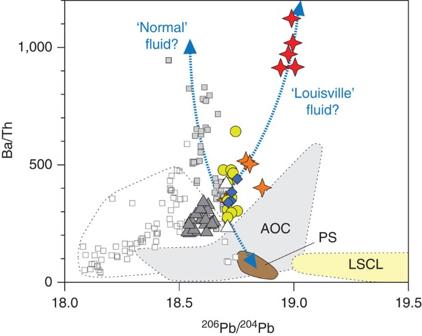Figure 4: Fluid composition. Ba/Th versus206Pb/204Pb modified after Turner and Hawkesworth63to determine the Pb isotope composition of the slab-derived ‘Louisville’ fluid. See caption ofFig. 3for data sources and acronyms. PS=Pelagic sediments. Figure 4: Fluid composition. Ba/Th versus 206 Pb/ 204 Pb modified after Turner and Hawkesworth [63] to determine the Pb isotope composition of the slab-derived ‘Louisville’ fluid. See caption of Fig. 3 for data sources and acronyms. PS=Pelagic sediments. Full size image Elevated 206 Pb/ 204 Pb and 208 Pb/ 204 Pb values in the northernmost Tonga arc volcanoes Tafahi and Niuatoputapu have been attributed to local Pb input from the subducted Louisville crust and volcaniclastics ( Fig. 1 ) (for example, refs 26 , 37 , 42 ). In contrast to the elevated 206 Pb/ 204 Pb and 208 Pb/ 204 Pb values in lavas from the central Tonga–Kermadec arc, those from Tafahi and Niuatoputapo are accompanied by higher 86 Sr/ 87 Sr, Th, Nb, Ta and light to middle rare-earth element contents, and low 143 Nd/ 144 Nd, interpreted to reflect a ~1% contribution of a sediment partial melt including a signature from the Louisville volcaniclastics [26] , [42] . However, ~2.5 to 14 Ma and 44 Ma lavas from Lau Ridge and Eua Island, which formed along the ‘proto Tonga-Kermadec’ (Vitiaz) arc, also display elevated 206 Pb/ 204 Pb, 208 Pb/ 204 Pb and 87 Sr/ 86 Sr, but higher 143 Nd/ 144 Nd values than the Niuatoputapu and Tafahi lavas (for example, refs 37 , 42 ). The elevated Lau Ridge 206 Pb/ 204 Pb and 208 Pb/ 204 Pb isotope signatures have therefore been present since ~44 Ma, suggesting that the high 206 Pb/ 204 Pb and 208 Pb/ 204 Pb isotope signatures represent a locally enriched mantle component beneath the northern Lau–Tonga Ridge system, likely introduced into the mantle beneath the northern-most Tonga arc system during the opening of the Lau Basin (for example, ref. 48 ). Furthermore, Todd et al. [41] suggests that these ambient mantle wedge compositional heterogeneities exist beneath the entire Tonga–Kermadec arc. The more extreme geochemical composition of the Tafahi and Niuatoputapu lavas could, therefore, be alternatively explained through partial melting of a locally enriched mantle with ocean-island-type affinities (± a sedimentary component), similar to the interpretation of Todd et al. [41] The lack of a Louisville signature in the lavas north of Ata suggests that such a signature can only be detected in more recent lavas in the vicinity of the subducting Louisville seamounts. There is uncertainty about the age of Ata Island but, based on moderate 238 U excess in Ata lavas and the lack of recent activity, it could be a few hundred thousand years old [26] . Similar to lavas from the central Tonga–Kermadec arc, back-arc lavas from the southern end of the Valu Fa ridge and Valu Fa off-axis seamounts located behind Ata Island have radiogenic 206 Pb/ 204 Pb and 208 Pb/ 204 Pb values ( Fig. 3a–d ) and elevated ratios of elements immobile in aqueous fluids (for example, (La/Sm) N ) (not shown) compared with mid-southern Lau basin lavas. The increases in 206 Pb/ 204 Pb, 208 Pb/ 204 Pb and (La/Sm) N strongly suggest regional-scale Louisville-related mantle source enrichment in proximity to the present intersection of the Louisville seamount chain with the Tonga–Kermadec trench. The alternative explanation for the elevated lava 206 Pb/ 204 Pb and 208 Pb/ 204 Pb values in the central Tonga–Kermadec arc lavas is ambient mantle heterogeneity [41] . However, partial melting of a heterogeneous mantle wedge would not only change fluid-mobile elements, but also fluid-immobile element ratios (such as La/Yb; Th/Yb, Zr/Y) and 143 Nd/ 144 Nd; although observed in Ata lavas, this is not observed in the lavas from Monowai, ‘U’ and ‘V’. A more westerly azimuth of the subducted Louisville seamount chain (see below), when combined with the observed isotopic anomaly in the lavas from the central Tonga–Kermadec arc system, strongly argues for a Louisville-derived signature, although the existence of an old, inherited enriched component in the mantle wedge beneath Ata cannot be ruled out. Location of the Louisville seamount chain beneath the arc Regionally, the Louisville collision zone is characterized by a 3 km shallowing in axial trench depth, a 15° anticlockwise rotation of the trench azimuth and a rough, hummocky forearc on the Indo-Australian plate. The small-scale morphological expressions of the Louisville collision zone can be isolated from the large-amplitude, long-wavelength trench-normal topographic expression of the Tonga–Kermadec subduction zone using spectral techniques ( Fig. 5 ). This long-wavelength signal often overwhelms and masks smaller-scale structures and when removed, residual bathymetric anomalies exceeding ±2 km are observed within the fore-arc, arc and back-arc of the Louisville collision zone ( Fig. 5 ). Positive bathymetric anomalies of ~2 km immediately NW of Osbourn seamount, the oldest (76.7±0.8 Ma) [49] unsubducted seamount in the Louisville chain, are interpreted as the presently subducting portion of the chain. Forearc bathymetric anomalies are, however, located west of the projected track of the Louisville seamount chain, assuming a continuation of the 340° azimuth observed on the seaward side of the trench. When coupled with bathymetric-positive anomalies observed along the southern portion of the Tonga Ridge and within the back-arc, a ~50° anticlockwise rotation in the geometry of the chain can be inferred. The elevated back-arc topography west to northwest of the contemporary collision zone has been attributed to underplating of Louisville Ridge crust [50] . 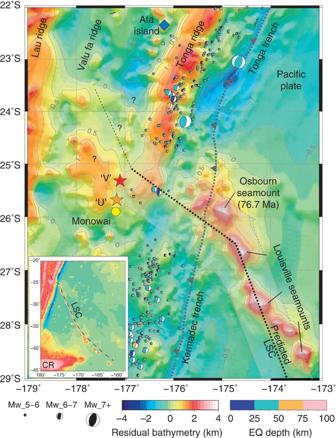Figure 5: Predicted Louisville hotspot track. Predicted Louisville hotspot track (black dashed line) reconstructed from absolute Pacific plate reconstruction rotations in model WK08-G by Wessel and Kroenke52(the location rotation point towards the westerly trend of the Louisville seamount chain south of Osbourn seamount is owing to the WK08-G models uncertainty). Grey lines provide 95% confidence region delimiting the maximum distance from the predicted track in which seamounts generated by the Louisville hotspot are observed. Grey dashed line with westward facing teeth demarcates the trench. Focal mechanisms for magnitudes ≥5 are from the Harvard CMT catalogue and are scaled according to magnitude and coloured for depth revealing the geometry of the Louisville seismic gap. CR, Chatham Rise; EQ, Earthquake; LSC, Louisville seamount chain; Mw, Earthquake Magnitude. Figure 5: Predicted Louisville hotspot track. Predicted Louisville hotspot track (black dashed line) reconstructed from absolute Pacific plate reconstruction rotations in model WK08-G by Wessel and Kroenke [52] (the location rotation point towards the westerly trend of the Louisville seamount chain south of Osbourn seamount is owing to the WK08-G models uncertainty). Grey lines provide 95% confidence region delimiting the maximum distance from the predicted track in which seamounts generated by the Louisville hotspot are observed. Grey dashed line with westward facing teeth demarcates the trench. Focal mechanisms for magnitudes ≥5 are from the Harvard CMT catalogue and are scaled according to magnitude and coloured for depth revealing the geometry of the Louisville seismic gap. CR, Chatham Rise; EQ, Earthquake; LSC, Louisville seamount chain; Mw, Earthquake Magnitude. Full size image The suggestion that the Louisville seamount chain has a more westerly track than its younger 340° azimuth is supported by another defining characteristic of the Louisville collision zone, namely, the region of seismic quiescence known as the ‘Louisville gap’ [51] ; Fig. 5 ). This gap shows a 40% reduction in shallow (0–100 km) seismicity compared with the regions immediately to the north and south, and the geometry of the sharp boundaries that delimit the seismic gap (when rotated 40–50° anticlockwise from the unsubducted Louisville seamount chain trend) supports an anticlockwise rotation in the geometry of the Louisville Ridge. The WK08-G total reconstruction rotation poles the Pacific plate of Wessel and Kroenke [52] suggest an anticlockwise rotation of ~35° for the Louisville seamount chain of seamounts about a point just to the south of Osbourn Seamount. The contemporaneity of the Osbourn Seamount (76.7±0.8 Ma) [49] with the Detroit seamount (75.8±0.6 Ma) [53] at the northern end of the Hawaii–Emperor seamount chain suggests that the anticlockwise kink in the Louisville seamount chain is the reciprocal of the Detroit–Meiji bend along the Emperor chain (for example, ref. 16 ) and can also be observed in the computed plume hotspot tracks of Steinberger et al. [54] An anticlockwise rotation in the subducted portion of the Louisville Ridge serves to limit the northward extent of paleo-ridge-collision zones and increases the age of collision between the Louisville Ridge and regions of the Tonga trench immediately north of the contemporary collision zone. Applying a 50° anticlockwise rotation for the portion of the Louisville seamount chain older than the Osbourn Seamount (76.7 Ma) in the kinematic model of Ruellan et al. [10] reduces the rate of southward migration of the intersection point of the seamount chain with the Tonga–Kermadec trench from ~180 km Myr −1 (ref. 20 , to <45 km Myr −1 ). Based on U-Th and 231 Pa- 235 U isotope data on lavas from Tonga–Kermadec arc-front volcanoes and the southern Lau Basin, it has been inferred that the time elapsed from fluid addition from the subducting slab to eruption was between ~30 kyr and 60 kyr (for example, refs 26 , 38 , 55 ). However, three studies on Tongan–Kermadec arc lavas estimated an even faster fluid addition time of <8 kyr [56] , [57] , [58] . Subduction recycling times of Pb are more difficult to obtain. It has been demonstrated [42] that Pb recycling times for slab-derived fluid addition to eruptions in the northern Tonga arc are between 0–3 Myr, with major fluid release occurring at 40–80 km depth during the transition from blueschist to eclogite, at temperatures of 500–600 °C (for example, refs 44 , 59 ). Assuming a constant convergence rate at the central Tonga–Kermadec arc of ~7 cm per year, the Louisville signature would require 0.6–1.2 Myr to reach the major fluid release zone at 40–80 km depth. In addition, assuming conservative 3 Myr for Pb from fluid addition to eruption as suggested by Regelous et al. [42] , the signature will require ~4 Myr from initial subduction to its appearance in the erupted lavas. Based on our revised southward migration of the Louisville collision zone of <45 km Myr −1 , the Louisville signature at ~40–80 km depth would have been located ~125 km further north than its present position (~180 km north of Monowai) ~3 Myr ago. This permits a maximum southward mantle flow of ~6 cm per year for the Louisville Pb isotopic signature to reach the source beneath the Monowai volcanic centre. However, as Pb is more fluid mobile than U (for example, [59] ) a significant proportion of Pb must have entered the melting zone within the past 50 kyr, as estimated by U-series disequilibria. Such fast recycling rates are consistent with a predominantly trench-normal mantle flow beneath the central Tonga–Kermadec arc. Elevated 206 Pb/ 204 Pb and 208 Pb/ 204 Pb in the lavas from Monowai to Ata are consistent with a lateral spread of the mantle containing a ~400 km-wide fluid-derived Louisville seamount chain component, suggesting either a laterally expanding and slightly southward moving mantle diaper, or the accretion of a flexurally supported and buoyant Louisville crust onto the forearc crust. This may also account for the more elevated topography of the arc north of the Louisville Ridge, compared with that to the south [10] . In addition, based on the revised southward migration rate of <45 km Myr −1 , initial subduction of the Louisville seamount chain must have occurred at least ~7 Myr ago to explain the geochemical anomaly in the lavas from Ata Island and the southern Valu Fa Ridge. Relatively stationary and continuous subduction of the Louisville chain for the past ~7 Myr, and possibly the under-plating of Louisville crust beneath the oceanic Australian Plate, can both explain the effective locking and cessation of back-arc opening rates south of the southern Lau Basin. Rapid southwards mantle flow has been proposed to occur beneath the northern Tonga arc and Lau Basin where back-arc opening rates are fast. Conversely, a threefold decrease in back-arc opening combined with the subduction underplating of Louisville crust may have resulted in greatly decelerated southward or trench-normal mantle flow beneath the central Tonga–Kermadec arc. Analytical details For trace element analysis, ~100 mg of powdered sample was digested in a microwave vessel using 6 ml of 28.9 M HF and 4 ml of 15.8 M HNO 3 . A 60-min ramped heat programme was run to 220 °C at a maximum of 40 bar. After completing the heating programme, the vessels were cooled to room temperature and carefully vented in a fume hood. After confirming complete sample digestion by visual inspection, evaporation was performed in two steps. The contents of each microwave vessel were quantitatively transferred to a Savillex digestion vessel, transferred to a 70 °C hotplate, and dried to incipient dryness to evaporate most of the HF and prevent fluoride formation. These vessels were allowed to cool, then 2 ml of 12.1 M HCl was added to each, which were then capped and heated to 150 °C on a hotplate for 24 h. The vessels were then allowed to cool, were uncapped and returned to a 70 °C hotplate to evaporate to incipient dryness. Finally, the residue was dissolved in 10 ml of 2 wt.% HNO 3 containing 1 p.p.b. In (internal standard) and made up to a final volume of 50 ml. Clear solutions were obtained in all cases and procedural blank solutions were also prepared. The solutions were analysed at the Queen’s Facility for Isotope Research, Kingston, Ontario, using an Element XR, High-Resolution inductively coupled plasma mass spectrometry (ICP-MS). Standard analyses are given in Supplementary Table S1 . Isotope analysis For chemical analysis, fresh cores of the samples were extracted, repeatedly washed in deionised water (in an ultrasonic bath) to remove sea salt, then crushed, handpicked and reduced to powder in an agate mill. Isotope analyses were undertaken at the University of Melbourne. Between 50 and 100 mg of fresh, clean chips, 1–5 mm in diameter, were handpicked for isotopic analysis and then leached in hot 6 N HCl for 30 min to remove any contaminants. Samples were then washed in ultrapure water and dissolved in HF/HNO 3 . Separation of Pb, Sr and Nd involved standard ion exchange procedures using Eichrom ion-specific resins. Analytical blanks are in all cases insignificant relative to the amount of sample processed and no blank corrections were made. Separated Sr, Nd and Pb were run on a Nu Instruments MC-ICP-MS using methods documented previously in Woodhead [60] for Pb and Hergt et al. [61] for Sr and Nd. 87 Sr/ 86 Sr was normalized to 86 Sr/ 88 Sr=0.1194 and reported relative to NIST SRM 987=0.710250. Internal precision is typically <0.000015 (2 s.e.) with reproducibility (2 s.d. of repeat runs) ≤±0.000040. 143 Nd/ 144 Nd was normalized to 146 Nd/ 145 Nd=2.0719425 (equivalent to 146 Nd/ 144 Nd=0.7219) and reported relative to La Jolla Nd=0.511865. Internal precision is typically <0.000010 (2 s.e.) with reproducibility (2 s.d. of repeat runs) ≤±0.000020. Pb isotope ratios are reported relative to SRM 981 values of 16.935, 15.489 and 36.701 with reproducibility (2 s.d. of repeat runs) ≤±0.03%. How to cite this article: Timm, C. et al. Louisville seamount subduction and its implication on mantle flow beneath the central Tonga–Kermadec arc. Nat. Commun. 4:1720 doi: 10.1038/ncomms2702 (2013).